Observation of conducting filament growth in nanoscale resistive memories Nanoscale resistive switching devices, sometimes termed memristors, have recently generated significant interest for memory, logic and neuromorphic applications. Resistive switching effects in dielectric-based devices are normally assumed to be caused by conducting filament formation across the electrodes, but the nature of the filaments and their growth dynamics remain controversial. Here we report direct transmission electron microscopy imaging, and structural and compositional analysis of the nanoscale conducting filaments. Through systematic ex - situ and in - situ transmission electron microscopy studies on devices under different programming conditions, we found that the filament growth can be dominated by cation transport in the dielectric film. Unexpectedly, two different growth modes were observed for the first time in materials with different microstructures. Regardless of the growth direction, the narrowest region of the filament was found to be near the dielectric/inert-electrode interface in these devices, suggesting that this region deserves particular attention for continued device optimization. Nanoscale resistive switching devices are typically based on two-terminal metal/insulator/metal (MIM) structures and have been extensively studied as a leading candidate for non-volatile memory [1] , [2] , [3] , [4] and reconfigurable logic [5] , [6] , [7] , [8] applications. Recently, they have also been linked to the concept of memristors [9] , [10] , [11] for analogue circuit [12] and neuromorphic computing [13] , [14] , [15] applications. For many devices, the resistive switching effect is believed to be caused by the formation of conducting filaments [16] , [17] , [18] , [19] , [20] , [21] . Understanding the dynamics of filament growth is thus of critical importance to continued device research. However, although the formation of conducting filaments has been visualized in several device systems [16] , [17] , [18] , [19] , these results only provided information of whether filaments exist or not in the on- and off-states. Questions crucial to device operation and optimization, such as where the filament begins to grow during programming and how the conducting channel is disconnected during erasing, remain unanswered. In addition, previous attempts to characterize conducting filaments were usually based on cross-sectional transmission electron microscopy (TEM) studies of pre-switched resistive memory devices [16] , [17] , [18] , [19] , where crucial filament regions may be missed during the sample-thinning process. The device is also completely destroyed after sample preparation, preventing detailed studies on filament dynamics from the same device. Recent attempts using in-situ TEM studies [20] , [21] have only focused on a small range of materials (mostly chalcogenide-based) without detailed analytical TEM characterizations. In this study, we provide unambiguous evidence that shows that localized, nanoscale filaments composed of elemental metals (and, in some cases, consisting of discrete nanoparticles instead of a solid wire) are formed during resistive switching. We found that the filament growth can be critically dependent on the cation mobility in the dielectric film, and report for the first time two different growth modes including a mode in which the conducting filament starts from the active electrode and grows towards the inert electrode, which was unexpected in theories developed for electrochemical metallization (ECM) memories [1] , [22] . The erasing mechanism was also studied by monitoring reverse growth of the filaments and the dielectric/inert electrode interface was found to be most important regardless of the filament growth directions, which was once again unexpected in previous hypotheses [22] , [23] . The growth dynamics and filament structures were systematically studied first for devices based on different switching materials in a lateral structure fabricated on ultrathin membranes (~15-nm-thick SiN x ). The results were further supported by in - situ TEM studies on memory devices with a vertical configuration. These findings, obtained from different material systems and from devices with different configurations, reveal several important and unexpected effects during filament growth and deserve particular attention in future device optimization. Ex - situ TEM on memory devices fabricated on SiN x membranes The devices consist of an active electrode and an inert electrode sandwiching a dielectric film in a lateral device structure, as schematically illustrated in the inset of Fig. 1a . These devices are based on metallic filament formation due to cation (for example, Ag or Cu ions) transport and redox processes and are sometimes termed ECM memories [22] , contrary to devices based on internal valence changes due to the redistribution of anions (for example, oxygen-ion diffusion for certain transition-metal oxide-based devices) [16] , [22] , [24] . In our studies, the active electrode and inert electrode are made of Ag and Pt, respectively. A wide range of materials, including main oxides (SiO 2 ), metal oxides (Al 2 O 3 ) and amorphous films (amorphous-silicon), have been used in this study as the dielectric layer in the MIM structure. These materials also possess different microstructures (from sputtered SiO 2 with high density of grain boundaries to amorphous silicon with densely packed clusters) and the results are representative of a large class of resistive switching devices using dielectrics as the switching layer. 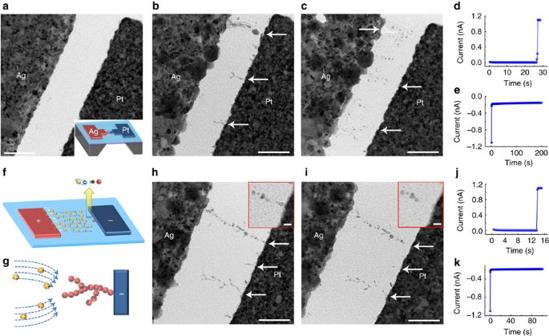Figure 1: Observation of conducting filament dynamics in SiO2-based resistive memories. (a) TEM image of an as-fabricated SiO2-based planar device fabricated on SiNxmembrane. Scale bar, 200 nm. Inset: schematic of the device. (b) TEM image of the same device after the forming process. The arrows highlight several representative filaments. Scale bar, 200 nm. (c) TEM image of the same device after erasing. Scale bar, 200 nm. (d) CorrespondingI–tcurve during the forming process that led to the image in (b). The applied voltage was 8 V. (e) CorrespondingI–tcurve during the erasing process that led to the image in (c). The applied voltage was −10 V. (f) Schematic of the filament growth process showing the transport and reduction of Ag cations. (g) Schematic of the dendrite structure formation. (h) TEM image of another device with a larger electrode spacing after the forming process. Scale bar, 200 nm. Inset: zoomed-in image of the filament (highlighted by the upper arrow) near the dielectric/inert electrode interface. Scale bar, 20 nm. (i) TEM image of the same device as in (h) after erasing. The dissolutions of the filaments were found to take place at the inert electrode interface. Scale bar, 200 nm. Inset: the same region as the inset in (h) after erasing. Scale bar, 20 nm. (j) CorrespondingI–tcurve during the forming process that led to the image in (h). The applied voltage was 10 V. (k) CorrespondingI–tcurve during the erasing process that led to the image in (i). The applied voltage was −10 V. Figure 1: Observation of conducting filament dynamics in SiO 2 -based resistive memories. ( a ) TEM image of an as-fabricated SiO 2 -based planar device fabricated on SiN x membrane. Scale bar, 200 nm. Inset: schematic of the device. ( b ) TEM image of the same device after the forming process. The arrows highlight several representative filaments. Scale bar, 200 nm. ( c ) TEM image of the same device after erasing. Scale bar, 200 nm. ( d ) Corresponding I – t curve during the forming process that led to the image in ( b ). The applied voltage was 8 V. ( e ) Corresponding I – t curve during the erasing process that led to the image in ( c ). The applied voltage was −10 V. ( f ) Schematic of the filament growth process showing the transport and reduction of Ag cations. ( g ) Schematic of the dendrite structure formation. ( h ) TEM image of another device with a larger electrode spacing after the forming process. Scale bar, 200 nm. Inset: zoomed-in image of the filament (highlighted by the upper arrow) near the dielectric/inert electrode interface. Scale bar, 20 nm. ( i ) TEM image of the same device as in ( h ) after erasing. The dissolutions of the filaments were found to take place at the inert electrode interface. Scale bar, 200 nm. Inset: the same region as the inset in ( h ) after erasing. Scale bar, 20 nm. ( j ) Corresponding I – t curve during the forming process that led to the image in ( h ). The applied voltage was 10 V. ( k ) Corresponding I – t curve during the erasing process that led to the image in ( i ). The applied voltage was −10 V. Full size image Figure 1a shows the TEM image of an as-fabricated device using sputtered SiO 2 as the dielectric layer. To switch the device, a constant positive voltage bias was applied to the Ag electrode with respect to the Pt electrode, and the current–time ( I – t ) characteristics were recorded as shown in Fig. 1d . The current remained very low until t ~26 s, when an abrupt increase in current was observed, implying that the device was turned into the on-state. This initial switching process is normally termed the forming process, and, for MIM devices, corresponds to the dissolution and injection of the active electrode material (for example, Ag) into the dielectric layer and formation of the initial filament [22] . Indeed, images taken after the forming process clearly revealed a well-defined conducting filament (highlighted by the top arrow in Fig. 1b ) with a typical conical shape. The filament is localized with a lateral size of ~20 nm near the tip and ~70 nm at the base, consistent with earlier findings and hypotheses [16] , [17] , [25] . Detailed TEM studies verified that the conducting filaments are composed of elemental Ag ( Supplementary Fig. S1 ), in agreement with the observations in ECM cells [1] , [22] . Besides the completed filament, a few incomplete filaments can also be clearly observed. The formation of a single dominant filament is consistent with the hypothesis that the filament formation is a self-limiting process, and, once a filament is completed, further filament growth will be suppressed owing to reduced electric field [26] . Of the over 100 devices studied, none showed more than one completed filament. More importantly, these studies reveal critical information about the dynamics of filament growth. Consistent with a well-established theory developed for ECM memories based on electrolytes [1] , [22] , the filaments in Fig. 1b apparently started growth from the inert electrode side as evidenced by the locations of the partially formed filaments. This can be explained by the reduction of the Ag cations at the negatively charged inert electrode side during the forming process [1] , [22] . Interestingly though, the cone shape of the filament in Fig. 1b is contrary to what is predicted by the ECM theory [1] , [22] . The thinnest part of the filament in Fig. 1b is apparently near the inert Pt electrode interface, with a much wider base formed near the active Ag electrode. Examination of the incomplete filaments also revealed similar geometry, with many of the incomplete filaments exhibiting a noteworthy dendrite structure with the branches pointing towards the active electrode (for example, the filament highlighted by the centre arrow in Fig. 1b ). In some sense, the cone structure for the complete filament in Fig. 1b can be thought of as a dendrite structure with the gaps between the branches also filled with Ag after the branches having reached the Ag electrode. Indeed, for devices with larger electrode spacings, dendrite-like filaments with branches pointing towards the active electrode, instead of cone-like filaments, were observed, as shown in Fig. 1h (highlighted by the upper arrow). It should be noted that the geometry of the filament is of fundamental importance in the operation of resistive memories because, during erasing/programming, the dissolution and recreation of the filaments are expected to occur at the thinnest part of the filament [23] . For ECM memories, this has been argued to be near the active electrode interface [23] , contrary to the findings here showing that the thinnest regions of the filaments are near the inert electrode interface instead (for example, Fig. 1b,h ). This observation leads to the suggestion that the dielectric/inert electrode interface, instead of the dielectric/active electrode interface, will be most critical during device operation for some dielectric-based devices. To verify this, we re-examined the devices after an erasing process, and subsequent TEM studies confirmed that the dissolution of the conducting filaments indeed occurs near the inert electrode interface. As shown in Figs 1c,i , all filaments, both completely formed and partially formed, were found to first break at the filament/inert electrode interface. When the erasing time is short ( Fig. 1k ), a narrow gap appears near the dielectric/inert electrode interface ( Fig. 1i and inset), whereas when the erasing time is long ( Fig. 1e ) sizable portions of the formed and partially formed filaments near the inert electrode interface are annihilated along with other visible nucleation sites ( Fig. 1c ). The dissolved parts of filaments were reversely deposited on the Ag side, as shown in Fig. 1c,i . It was found that the filaments were rarely fully dissolved. As shown in Fig. 1i , after the initial rupture of the filament at the narrowest region near the filament/inert electrode interface, the rest of the filament is no longer electrically connected to the positively biased inert electrode, resulting in less-efficient redox processes. As a result, a substantial number of filament materials may still exist in the dielectric film after erasing, and can facilitate subsequent filament growth. This effect explains the observations in ECM devices that lower threshold voltages are typically required during programming processes, compared with those for the initial forming process [22] , [27] , [28] . The differences between the results reported here and the theory based on chalcogenide-based ECM cells are noteworthy, because understanding which interface dominates the filament formation/dissolution process is of high importance for continued device optimizations. We believe that these differences highlight the critical role of cation transport during resistive switching. For chalcogenides such as GeS x and GeSe x , which are Ag electrolytes with high cation mobility, the programming process is accompanied by a large ionic current caused by a large volume of Ag cations moving through the electrolyte and being reduced at the inert cathode, resulting in a reverse cone-shaped filament growing backwards towards the active electrode [1] , [22] . On the other hand, for devices based on dielectrics that are not typical electrolytes (such as SiO 2 and other oxides) the growth of the filament can be limited by the cation supply instead. As shown schematically in Fig. 1f,g , the filament still initiates from the inert electrode ( Fig. 1f ), but, during subsequent growth, the limited amount of cations will preferably diffuse to and become reduced at the end of the existing filament, because the front of the protrusion will have the highest electric field. This process in turn creates a branched growth with the dendrites pointing towards the active electrode as determined by the distorted electric field lines ( Fig. 1g ). As a result, the region near the dielectric/inert electrode interface will have the narrowest filament and thus will be most critical during device operations for these dielectric-based devices. It should be noted that a prerequisite for the observation of such dendrite structures is that the cation transport is the dominant rate-limiting process during filament growth, which poses an upper limit on the cation concentration. In contrast, in the case of high cation concentrations such as in solid electrolyte (for example, chalcogenide)-based devices, the reduction of cations and the crystallization of filaments will require significant space expansion [27] , and the reduction/crystallization process can become the rate-limiting process. As a result, in those cases, most of the cations will reach the inert electrode and be reduced there, resulting in conducting filaments with their bases at the dielectric/inert electrode interface. To further illustrate the role of cation transport in dielectric-based resistive memories, other materials such as atomic layer deposition (ALD)-prepared Al 2 O 3 and plasma-enhanced chemical vapour deposition (PECVD)-grown amorphous silicon (a-Si) were also studied as the I-layer in MIM device structures. Similar results were obtained from Al 2 O 3 films ( Supplementary Fig. S2 ) because both ALD Al 2 O 3 and sputtered SiO 2 contain a high density of defects and offer similar diffusion paths for cation transport. On the other hand, further information was obtained when examining PECVD-grown a-Si-based devices, which provides even lower cation mobility owing to the densely packed Si clusters. First we noticed that a-Si-based MIM devices require much longer time and higher electric field to be formed compared with sputtered SiO 2 -based devices, consistent with the lower cation mobility argument. More interestingly, studies on these devices suggest that not only the filament shape but also its growth direction can be affected by cation mobility. 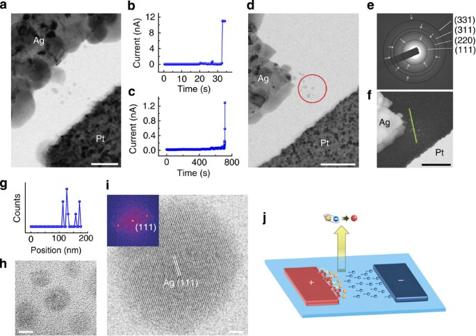Figure 2: Observation of conducting filament dynamics in amorphous-Si-based resistive memories. (a) TEM image of a complete conducting filament in an a-Si-based device. The thinnest region of the filament is at the dielectric/inert electrode interface. Scale bar, 50 nm. (b) The correspondingI–tcurve for device in (a) during the forming process. The applied voltage was 8 V. (c)I–tcurve for another device in (d) during the forming process. The applied voltage was 10 V. (d) TEM image of the device showing a partially formed filament. The filament apparently grew from the active electrode. The region indicated by the red circle was analysed by SAED. Scale bar, 100 nm. (e) SAED pattern of the filament indexed with elemental Ag with fcc structure. (f)Z-contrast HAADF STEM image of the filament. Scale bar, 100 nm. The green line indicates the position for EDS line profile analysis. (g) Corresponding EDS line profile results showing the Ag signal intensity. (h) HRTEM image showing a group of nanoparticles inside the filament. Scale bar, 2 nm. (i) Bright-field STEM image of a Ag nanoparticle in the conducting filament. The lattice fringes were indexed to the Ag fcc structure. Scale bar, 2 nm. Inset: corresponding fast Fourier transformation results of the HRTEM image. (j) Schematic of the filament growth for a-Si-based resistive memories showing that the cations can be reduced inside the dielectric film by free electrons. Figure 2a shows the TEM image of a complete filament in the a-Si-based devices. The accompanying I – t forming curve is shown in Fig. 2b . Here again, a cone-shaped structure was observed with the wide base near the active Ag electrode and the narrow neck near the inert Pt electrode. Similarly shaped filaments were observed in many other devices (for example, Fig. 3h ). Furthermore, by using a lower programming current ( Fig. 2c ), a partially formed filament can be obtained as shown in the TEM image Fig. 2d . Surprisingly, here the filament seems to start growing from the active Ag electrode (anode) instead. This effect is completely unexpected in the conventional ECM theory as the cations are supposed to reach the negatively charged cathode side (either the inert electrode or protrusions grown from it, for example, partially formed filaments in Fig. 1 ) to be reduced, and elemental metal-based filaments theoretically cannot exist without this reduction process. To uncover the nature of the observed filaments, such as their compositions and chemical states, detailed material characterizations were performed through analytical TEM. The crystal structure of the partially formed filament was studied by selected area electron diffraction (SAED), and the region of interest is marked by the red circle in Fig. 2d . The diffraction spots in the SAED pattern can be successfully indexed to the elemental phase of Ag with a face-centred cubic (fcc) structure ( Fig. 2e ), demonstrating that the filament is indeed composed of metallic elemental Ag. Because both the switching medium (a-Si) and the supporting SiN x membrane underneath are amorphous in nature, they appear as diffusive haloes in the SAED pattern. Figure 2f shows a Z -contrast high-angle annular dark-field (HAADF) scanning transmission electron microscopy (STEM) image of the filament. The filament composition was further analysed by energy-dispersive X-ray spectroscopy (EDS) in STEM mode ( Supplementary Fig. S3 ) and line profile analysis ( Fig. 2g ) along the green line in Fig. 2f , again revealing clear Ag signals along the conducting pathway. Figure 2h presents a high-resolution TEM (HRTEM) image of the conducting filament, where the filament is found to be composed of a series of Ag nanoparticles separated by gaps of nanometer scale (ranging from 1 to 4 nm in Fig. 2h ). These nanoscale gaps will allow efficient electron tunnelling so that the conducting filament can still offer conductance in the on-state, even though it is composed of a chain of nanoparticles instead of a solid wire. Figure 2i shows a representative bright-field STEM image of a Ag particle inside the filament. The lattice fringes could be successfully indexed with (111) crystal planes of fcc Ag, in agreement with the SAED results. The corresponding fast Fourier transformation also verifies that the Ag particle is elemental Ag with fcc structure (inset). Figure 2: Observation of conducting filament dynamics in amorphous-Si-based resistive memories. ( a ) TEM image of a complete conducting filament in an a-Si-based device. The thinnest region of the filament is at the dielectric/inert electrode interface. Scale bar, 50 nm. ( b ) The corresponding I – t curve for device in ( a ) during the forming process. The applied voltage was 8 V. ( c ) I – t curve for another device in ( d ) during the forming process. The applied voltage was 10 V. ( d ) TEM image of the device showing a partially formed filament. The filament apparently grew from the active electrode. The region indicated by the red circle was analysed by SAED. Scale bar, 100 nm. ( e ) SAED pattern of the filament indexed with elemental Ag with fcc structure. ( f ) Z -contrast HAADF STEM image of the filament. Scale bar, 100 nm. The green line indicates the position for EDS line profile analysis. ( g ) Corresponding EDS line profile results showing the Ag signal intensity. ( h ) HRTEM image showing a group of nanoparticles inside the filament. Scale bar, 2 nm. ( i ) Bright-field STEM image of a Ag nanoparticle in the conducting filament. The lattice fringes were indexed to the Ag fcc structure. Scale bar, 2 nm. Inset: corresponding fast Fourier transformation results of the HRTEM image. ( j ) Schematic of the filament growth for a-Si-based resistive memories showing that the cations can be reduced inside the dielectric film by free electrons. 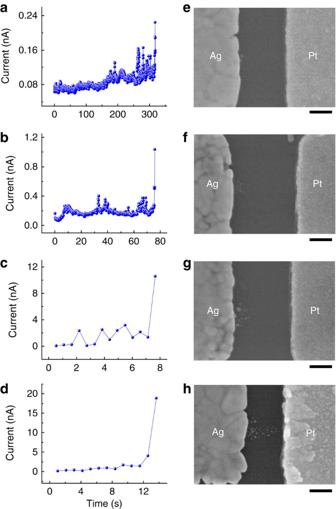Figure 3: Controlling the filament size by limiting the programming current. (a–d)I–tcurves with different programming currents during the forming process and (e–h) corresponding SEM images of the devices after forming, showing the correlation of the filament size with the programming current. Scale bar, 100 nm. Four different a-Si-based devices with similar geometry were used in this study. The applied voltages were (a) 18 V, (b) 26 V, (c) 22 V, and (d) 20 V, respectively. Full size image Figure 3: Controlling the filament size by limiting the programming current. ( a – d ) I – t curves with different programming currents during the forming process and ( e – h ) corresponding SEM images of the devices after forming, showing the correlation of the filament size with the programming current. Scale bar, 100 nm. Four different a-Si-based devices with similar geometry were used in this study. The applied voltages were ( a ) 18 V, ( b ) 26 V, ( c ) 22 V, and ( d ) 20 V, respectively. Full size image These examinations unambiguously reveal that Ag cations can indeed be reduced inside the dielectric without reaching the cathode, resulting in conducting filaments growing from the active electrode side in dielectric-based resistive memories with low cation mobility. The main question now is how the reduction process occurs and where the negative charges come from to reduce the cations. In Ag electrolytes (that is, chalcogenides such as GeS x or GeSe x ) with high cation mobility, Ag ions reach the cathode very quickly and become reduced there [22] , [29] . However, in dielectrics that offer very low cation mobility, the Ag ions move much more slowly and the cation transport can become the rate-limiting process, leading to possible reduction of Ag ions inside the dielectric by capturing free electrons injected from the cathode, as schematically shown in Fig. 2j . It should be noted that the introduction of Ag cations into the dielectric should clearly obey general electroneutrality conditions and, therefore, the cations must be balanced by electrons injected from the counter electrode with the same flux rate. In fact, it has been calculated that even for dielectrics with high cation mobility the main contribution to the programming current is still the electronic current instead of the ionic current, [30] so reduction through the electron current is clearly a possibility. Whether the cations are reduced inside the dielectric or at the cathode then depends on the rate-limiting factor of the various thermodynamic processes [22] in specific systems. For example, for sputtered defective SiO 2 , where the Ag ions can diffuse relatively fast, most cations will be reduced when they reach the negatively charged cathode side, as schematically illustrated in Fig. 1g , whereas for PECVD-grown amorphous silicon the densely packed clusters result in very low cation mobility and Ag cations may only travel a short distance inside the dielectric before they are reduced by capturing incoming free electrons, as schematically illustrated in Fig. 2j . In this case, the Ag precipitates are formed near the anode and will serve as an extension of it. The repeated ionization, short-distance transport and reduction processes ( Supplementary Fig. S4 ) lead to filament growth from the active electrode (anode) towards the inert electrode (cathode) during programming, as verified experimentally in Figs 2 and 3 and Supplementary Fig. S5 . These findings in turn suggest that the dynamics of filament growth in dielectric-based resistive memories can be critically limited by the ion transport process in the switching medium, more so as compared with electrochemical reactions occurring at the electrodes. Detailed analysis of the electrochemical processes and cation transport dynamics during filament growth are subject to further investigations. These arguments also predict that it is possible to control the filament growth by adjusting the programming current. As shown in Fig. 3 , four different devices with similar structures were programmed with different programming currents ( Fig. 3a–d ), and an increase of the programming current indeed resulted in an increase in filament size, both in length and in width ( Fig. 3e–h ). Similar effects were also observed from a single device, as shown in Supplementary Fig. S5 , where the application of a second programming process led to an extension of the existing filament towards the inert electrode, illustrating the possibility of step-by-step growth of the filament from the active electrode to the inert electrode in these devices. These results indicate that the growth of filaments is impacted by the electron current, and are consistent with the picture that the Ag ions are reduced inside dielectrics by capturing free electrons. The filament growth dynamics was further studied by examining the wait time before the sharp resistance-switching event (denoted as t w ) as a function of electric field and temperature, respectively. In general, the filament growth is determined by three dynamic processes [27] : (i) the anodic dissolution of the metal component at the active electrode; (ii) the transport of the metal ions through the dielectrics; and (iii) the reduction of metal ions and the crystallization of conducting filaments. All these three stages can potentially be the rate-limiting process in ECM cells. Our studies on different dielectrics-based devices show that the switching behaviours (switching time, electric field required and growth direction) are significantly influenced by the choice of dielectrics ( Figs 1 , 2 , 3 , Supplementary Figs S2, S6 and S7 ). Therefore, the electrochemical dissolution of the active electrode and the reduction/nucleation of the cations, which are not strongly dependent on the choice of dielectrics, are likely not the rate-limiting processes here. As the cation transport process is completely inside the dielectric film and strongly dependent on the dielectric properties, it is reasonable to conclude that the cation transport process is the rate-limiting process for devices studied here, especially for dielectrics with low cation mobility. 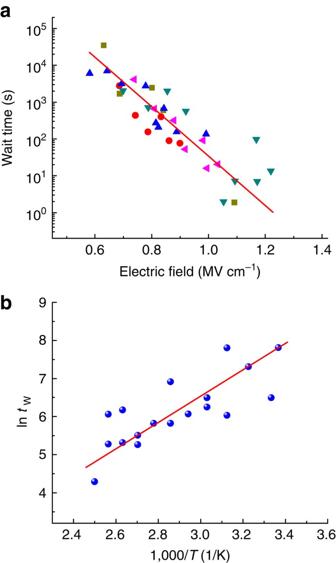Figure 4: Electric field and temperature dependence of the wait time. (a) Wait time as a function of the applied electric field for devices with various electrode spacingd.The different symbols of square, circle, upper triangle, lower triangle, and left triangle correspond todvalues of 70–195, 195–215, 250–270, 280–305, and 320–355 nm, respectively. Results from 36 a-Si-based resistive switches were presented. (b) Arrhenius plot of the wait time as a function of temperature under a constant electric field of 0.8 MV cm−1. Figure 4a shows the electric field dependence of t w for a large number of a-Si-based devices with a wide range of electrode spacing d , ranging from 70 to 355 nm. Here the electric field E is defined by E = V/d , where V is the applied voltage bias. It is evident from Fig. 4a that all data obtained from different devices collapse into a single curve when plotted against the electric field. This universal scaling curve further verifies that the filament growth is facilitated by the electric field, in agreement with the hypothesis of field-assisted ion transport inside the dielectric [31] , [32] . During ion transport, the activation energy E a ′ seen by the ion will be lowered to first order by a term linearly dependent on the electric field [31] , [32] , E a ′ = E a − aE . The average wait time, as a statistical quantity, is then determined by: Figure 4: Electric field and temperature dependence of the wait time. ( a ) Wait time as a function of the applied electric field for devices with various electrode spacing d. The different symbols of square, circle, upper triangle, lower triangle, and left triangle correspond to d values of 70–195, 195–215, 250–270, 280–305, and 320–355 nm, respectively. Results from 36 a-Si-based resistive switches were presented. ( b ) Arrhenius plot of the wait time as a function of temperature under a constant electric field of 0.8 MV cm −1 . Full size image where is the attempt frequency, k B is the Boltzmann constant and T is the absolute temperature. Equation (1) suggests that the wait time will be reduced exponentially as a function of the electric field, consistent with the data shown in Fig. 4a . For comparison, Fig. 4b plots t w as a function of temperature under a constant electric field of 0.8 MV cm −1 . The curve can be fitted to an Arrhenius plot with a general relationship of ln t 1/T , again consistent with equation (1) and supports the picture that filament formation is dominated by the cation transport process in these dielectric-based resistive memories. In - situ TEM studies on vertical device structures The proposed picture of filament growth was further verified in devices with a vertical configuration via in - situ TEM observations. The memory device was fabricated on a W probe by depositing a conformal PECVD a-Si film layer, and the MIM structure was formed when the W probe with the dielectric layer was brought in contact with a high-purity Ag wire to form the W/a-Si/Ag structure shown in Fig. 5a . During device operation, external voltage biases were applied to the Ag electrode with respect to the W electrode, and the device was imaged inside a TEM chamber while the I – t curves were recorded. The conformal coating of the a-Si film over the W probe assures that the filament has to penetrate the bulk of the a-Si layer before electrical connection between the Ag and W probes can be created. Detailed specimen preparation and manipulation approaches can be found in Methods. 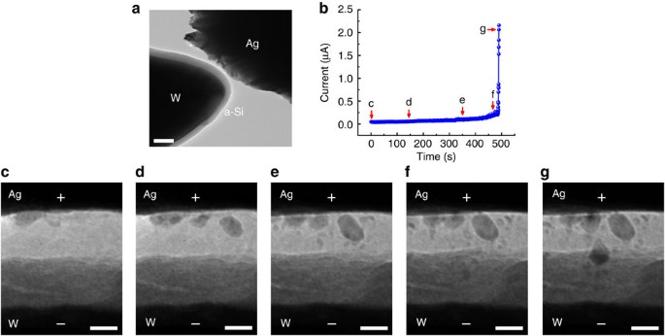Figure 5:In-situTEM observation of conducting filament growth in vertical Ag/a-Si/W memories. (a) Experimental set-up. The Ag/a-Si/W resistive memory device was fabricated on a W probe. Scale bar, 100 nm. (b)I–tcharacteristics recorded during the forming process at a voltage of 12 V. (c–g) TEM images of the device corresponding to data points c–g in (b) recorded during the forming process. Scale bar, 20 nm. Figure 5b displays the I – t characteristics during the forming process; a clear resistance switching event from the pristine high-resistance state to the low-resistance state was observed at ~490 s. During switching, the filament growth process was directly observed in real time and recorded by a digital camera ( Supplementary Movie 1 ). Figure 5c–g plots the representative TEM images of the device at different switching stages, corresponding to points c–g in Fig. 5b . Once again the filament growth was found to initiate from the active electrode ( Fig. 5d ), and the filament features a conical shape with the broadest base at the active Ag electrode side ( Fig. 5g ), in agreement with the findings from ex-situ TEM studies. Moreover, these images reveal that the base, grown from the active electrode ( Fig. 5d ), serves as a reservoir of the metal ions for subsequent growth; while discrete metal particles are created subsequently as the filament is extended towards the inert electrode, as shown in Fig. 5e–g . Similarly, in-situ TEM studies on the erasing process of an already-programmed device show that filament dissolution is initiated from the filament/inert electrode interface, and the filament material is re-deposited towards the active electrode as the device is erased ( Supplementary Fig. S8 ). These in-situ TEM results unambiguously verify the conclusions obtained from the ex-situ TEM studies: that is, that filament growth can be initiated from the active electrode and that filament retraction can start from the filament/inert-electrode interface, which are behaviours that were unexpected from existing ECM theory developed for electrolyte-based devices. Figure 5: In - situ TEM observation of conducting filament growth in vertical Ag/a-Si/W memories. ( a ) Experimental set-up. The Ag/a-Si/W resistive memory device was fabricated on a W probe. Scale bar, 100 nm. ( b ) I – t characteristics recorded during the forming process at a voltage of 12 V. ( c – g ) TEM images of the device corresponding to data points c–g in ( b ) recorded during the forming process. Scale bar, 20 nm. Full size image The formation and evolution of nanoscale conducting filaments in resistive memories have been systematically studied in different material systems and device configurations, and it was found that filament growth can be limited by the cation transport process, and two different growth modes can occur. In both cases, however, the narrowest region of the filament was found to be near the dielectric/inert-electrode interface, suggesting the importance of this region in continued device optimization. These studies will broaden our understanding of the switching mechanism in filament-based resistive memories and will stimulate continued material and device optimizations of this important class of devices. We also note that the switching time and the electric field used in these studies are still different from the conditions of standard ECM cell operations, and the filament growth for a specific device under specific operation conditions will be determined by the interplay of different filament growth dynamics [1] , [22] and needs to be analysed individually. Fabrication of planar resistive switches on SiN x membrane The low-stress SiN x membranes were purchased from Ted Pella. The SiN x membranes have a small thickness of 15 nm and produce a low background under TEM. The active dielectric layer thickness was also kept low at ~15 nm to further improve the electron transparency of the devices. The electrodes were fabricated by electron beam lithography (Raith 150) followed by electron beam evaporation and lift-off processes. A two-step lithography process was employed. The 25-nm Pt electrode with a 5-nm Ti adhesion was fabricated first, followed by the Ag electrode alignment, patterning, and lift-off (thickness ~40 nm). Special care was taken when handling the fragile and small SiN x membranes during the multiple steps of fabrication process. Similar device structures were also fabricated on Si/SiO 2 substrates for scanning electron microscopy (SEM) studies. The use of ultrathin membranes in a lateral device makes it possible to directly image any structural changes down to very small scales. Compared with previous attempts [16] , [17] , [18] , [19] , this approach also guarantees the observation of all filaments (formed or partially formed) and allows direct study on the evolution of the same filaments at different programming and erase conditions. To minimize possible e-beam damage to the device during the filament formation process, the devices were programmed in a separate controlled environment and only exposed to high-energy electrons after the filament evolution has been completed. Switching dielectrics deposition Three types of films with a thickness of ~15 nm were deposited as the switching dielectrics: SiO 2 , Al 2 O 3 , and a-Si. The SiO 2 films were deposited either by radio frequency sputtering at room temperature ( Fig. 1 and supplementary Fig. S6 ) or in a thermal furnace ( Supplementary Fig. S7 ). The Al 2 O 3 films were deposited by ALD (Oxford OpAL) using a thermal ALD process, and trimethylaluminum and H 2 O as precursors, at 150 °C. The a-Si films were deposited by plasma-enhanced chemical vapour deposition (GSI UltraDep 2000) at 350–400 °C. Electron microscopy The STEM images were obtained in a C s -corrected JEOL 2100F TEM by a HAADF detector at an accelerating voltage of 200 kV. The HRTEM observations and SAED characterizations were conducted in a JEOL 3011 (300 kV) and a JEOL 2010F (200 kV) TEM. The EDS analyses were performed in a JEOL 2010F TEM. The in - situ TEM experiments were carried out in the JEOL 3011 TEM. Two scanning electron microscopes were used in SEM characterizations at accelerating voltages of 10–15 kV: FEI Nova Nanolab and Hitachi SU8000. Electrical measurements Electrical measurements for ex-situ studies were performed using a low-noise Keithley 4200 semiconductor characterization system combined with a probe station (Desert Cryogenics TTP4), while the measurements for in-situ studies were performed by Keithley 4200 combined with a Nanofactory system. Current compliance was applied to protect the devices and to control the filament size. The temperature of the sample holder of the probe station can be varied by a temperature controller (Lakeshore 332) for temperature-dependent studies. To reduce the effect of heating, low-programming currents ~10 nA were used in ex - situ measurements. As relatively wider gaps were used in the lateral devices (~100 nm compared with <50 nm used in vertical devices), a higher programming voltage is needed to provide the required electric field for filament formation. We note that since the current compliance is supplied externally, some current overshoot is likely and the level of current overshoot is amplified with increased voltage. As a result, keeping the programming current compliance low is critical to allow the formation of nanoscale filaments. All images shown in the ex - situ studies were taken individually after the filament had been programmed/erased to minimize possible e-beam damage to the device during the filament formation process. In - situ TEM The in - situ TEM specimen was prepared by depositing a conformal a-Si film on a W probe (Bruker) with a PECVD process. The W probe was then mounted on the moveable end of a single-tilt TEM holder. A high-purity Ag wire (99.99%, Goodfellow) was fixed on the other end of the TEM holder to serve as the active electrode. The movement of the W probes was controlled by a Nanofactory system to achieve contact with the Ag wire, forming a Ag/a-Si/W memory structure. During in - situ experiments, the electron beam current was kept low (<1 fA/nm 2 ) to minimize e-beam damage. How to cite this article: Yang, Y. et al . Observation of conducting filament growth in nanoscale resistive memories. Nat. Commun. 3:732 doi: 10.1038/ncomms1737 (2012).